Quantum simulation of low-temperature metallic liquid hydrogen The melting temperature of solid hydrogen drops with pressure above ~65 GPa, suggesting that a liquid state might exist at low temperatures. It has also been suggested that this low-temperature liquid state might be non-molecular and metallic, although evidence for such behaviour is lacking. Here we report results for hydrogen at high pressures using ab initio methods, which include a description of the quantum motion of the protons. We determine the melting temperature as a function of pressure and find an atomic solid phase from 500 to 800 GPa, which melts at <200 K. Beyond this and up to 1,200 GPa, a metallic atomic liquid is stable at temperatures as low as 50 K. The quantum motion of the protons is critical to the low melting temperature reported, as simulations with classical nuclei lead to considerably higher melting temperatures of ~300 K across the entire pressure range considered. Ever since Wigner and Huntington’s prediction in 1935 that solid molecular hydrogen would dissociate and form an atomic and metallic phase at high pressures [1] , the phase diagram of hydrogen has been the focus of intense experimental and theoretical studies [2] , [3] , [4] , [5] , [6] , [7] . Advanced experimental techniques, notably diamond anvil cell approaches, mean that it is now possible to explore hydrogen at pressures up to about 360 GPa [2] , [8] , [9] , [10] , and new types of diamond anvil cell may be able to access much higher pressures [11] . These experiments, along with numerous theoretical studies, have revealed a remarkably rich and interesting phase diagram comprising regions of stability for a molecular solid, a molecular liquid and an atomic liquid, and within the solid region four distinct phases have been detected [9] , [10] , [12] , [13] . Furthermore, metallic hydrogen has been observed in high-temperature shock-wave experiments [14] , [15] and it is accepted to be a major component of gas giant planets, such as Jupiter and Saturn [15] . Despite the tremendous and rapid progress, important gaps in our understanding of the phase diagram of high-pressure hydrogen remain, with arguably the least well-understood issue being the solid to liquid melting transition at very high pressures. Indeed the melting curve is only established experimentally and theoretically up to around 200 GPa [5] , [6] . However, from 65 GPa up to about 200 GPa, the slope of the melting curve is negative (that is, the melting point drops with increasing pressure), which suggests that at yet higher pressures a low temperature liquid state of hydrogen might exist or, as suggested by Ashcroft [16] , perhaps even a metallic liquid state at zero K. Further interest in hydrogen at pressures well above 200 GPa stems from other remarkable suggestions, such as superfluidity [4] and superconductivity at room temperature [17] , [18] , all of which imply that hydrogen at extreme pressures could be one of the most interesting and exotic materials in all of condensed matter. In the current study we use computer simulation techniques to probe the low-temperature phase diagram of hydrogen in the ultra-high 500–1,200 GPa regime to try and find this potential low-temperature liquid state of hydrogen. We describe the proton motion using ab initio path-integral molecular dynamics (PIMD) methods [19] , [20] , [21] , [22] , [23] , [24] , which are based on electronic structures computed ‘on the fly’ as the dynamics of the system evolves, and can account for bond formation and breaking in a seamless manner. To compute the melting curve we simulate solid and liquid phases in coexistence [5] , [25] , [26] . The coexistence approach minimizes hysteresis effects arising from superheating or supercooling during the phase transition, and although it has been used with model potentials and ab initio approaches before the current study is, to the best of our knowledge, the first to combine it with the ab initio PIMD method. This treatment amounts to considering the Gibbs free energy of the liquid and solid phases when calculating the melting curve. With this combination of approaches we have found a low-temperature metallic atomic liquid phase at pressures of 900 GPa and above, down to the lowest temperature we can simulate reliably of 50 K. The existence of this low-temperature metallic atomic liquid is associated with a negative slope of the melting curve between atomic liquid and solid phases at pressures between 500 and 800 GPa. This low-temperature metallic atomic liquid is strongly quantum in nature, as treating the nuclei as classical particles using the ab initio molecular dynamics (MD) method significantly raises the melting curve of the atomic solid to ~300 K over the whole pressure range. The classical treatment of the nuclei does not reproduce a notable negative slope of the melting curve, and consequently does not predict a low-temperature liquid phase. Our study provides a finite temperature phase diagram of hydrogen under ultra-high pressures and gives direct numerical support for Ashcroft’s low-temperature metallic liquid. Two-phase simulations with PIMD Extensive computational searches for low-enthalpy solid structures of hydrogen have been performed using density functional theory methods [27] , [28] , [29] , [30] , [31] , and recently a systematic analysis of the evolution of the low-enthalpy phases has been provided by Labet et al. [32] , [33] . These searches found a metallic phase of I 4 1 / amd space group symmetry to be stable from about 500 to 1,200 GPa (ref. 30 ), when quasi-harmonic proton zero-point motion was included. We use this phase, therefore, as the starting point for our finite temperature exploration of the phase diagram and melting curve. With the coexistence method, we have performed a series of two-phase solid–liquid simulations at different temperatures (from 50 to 300 K), which are then used to bracket the melting temperature from above and below. We begin by considering the 500–800 GPa pressure regime and show an example of the data obtained from the coexistence simulations at 700 GPa in Fig. 1 . At this pressure we find that for T ≥125 K, the system transforms into a liquid state, whereas for T ≤100 K, it ends up as solid. To characterize these states, we have used a pair-distribution function and averaged out its angular dependence. The result is a function of interatomic separations, which is denoted by g ( r ) throughout this manuscript. In a liquid, this is the so-called radial distribution function. As can be seen in Fig. 1d , upon moving from 100 to 125 K the system clearly possesses less structure, indicating that a transition from solid to liquid occurs. These phases were also characterized by the variations in mean square displacement of the nuclei of the particles over time. As PIMD rigorously provides only thermally averaged information, we used the adiabatic centroid MD approach within the path-integral scheme to obtain real-time quantum dynamical information [34] . Again, as shown in Fig. 1e , the distinction between the solid phase at 100 K and liquid phase at 125 K is clear. 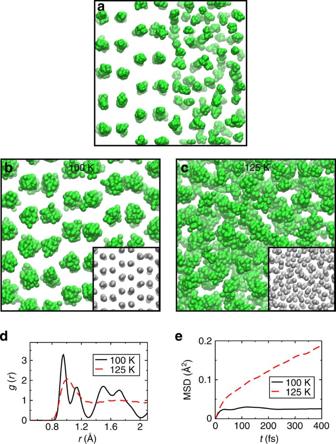Figure 1:Ab initioPIMD simulations of solid–liquid coexistence and melting. Snapshots of the PIMD simulations at 700 GPa showing (a) the starting structure, (b) the final state at 100 K and (c) the final state at 125 K. Thirty-two beads (green balls) were used to represent the imaginary-time path integral for each atom. The grey balls in the insets ofbandccorrespond to the centroid of each atom. (d) The angularly averaged pair-distribution functiong(r) for the same two simulations at 100 and 125 K. At 100 K, the solid state persists (black solid line) as indicated by the relatively sharp peaks. At 125 K (red dashed line), these peaks are much broader and theg(r) is characteristic of a liquid. This is further supported by the data ine, where the mean square displacements (MSD) as a function of time from separate adiabatic centroid MD simulations within the path-integral framework are shown34. The MSD for the 100 K solid phase saturates rapidly, whereas for the liquid phase at 125 K it rises approximately linearly with time, resulting in a finite diffusion coefficient. Figure 1: Ab initio PIMD simulations of solid–liquid coexistence and melting. Snapshots of the PIMD simulations at 700 GPa showing ( a ) the starting structure, ( b ) the final state at 100 K and ( c ) the final state at 125 K. Thirty-two beads (green balls) were used to represent the imaginary-time path integral for each atom. The grey balls in the insets of b and c correspond to the centroid of each atom. ( d ) The angularly averaged pair-distribution function g ( r ) for the same two simulations at 100 and 125 K. At 100 K, the solid state persists (black solid line) as indicated by the relatively sharp peaks. At 125 K (red dashed line), these peaks are much broader and the g ( r ) is characteristic of a liquid. This is further supported by the data in e , where the mean square displacements (MSD) as a function of time from separate adiabatic centroid MD simulations within the path-integral framework are shown [34] . The MSD for the 100 K solid phase saturates rapidly, whereas for the liquid phase at 125 K it rises approximately linearly with time, resulting in a finite diffusion coefficient. Full size image Melting curve and the low-temperature metallic liquid The same coexistence procedure was used to locate the melting point at 500 and 800 GPa, leading to the melting curve shown in Fig. 2 . The up (down) triangles indicate the highest (lowest) temperatures at which the solid (liquid) phases are stable, bracketing the melting temperatures within a 25-K window. From this we see that the melting temperature is 150–175 K at 500 GPa, and that it drops rapidly with increasing pressure, yielding a melting temperature of only 75–100 K at 800 GPa. Thus, the melting curve has a substantial negative slope ( dP / dT <0) in this pressure range. Across this entire pressure range the molten liquid state is atomic, and the solid phase, which grows, is the original atomic I 4 1 / amd phase that was used as the starting structure. Given that molecular phases have been observed at pressures lower than 360 GPa in both experimental and theoretical studies [8] , [10] , we suggest that a molecular-to-atomic solid–solid phase transition should occur between 360 GPa and the lowest pressure of 500 GPa considered here. 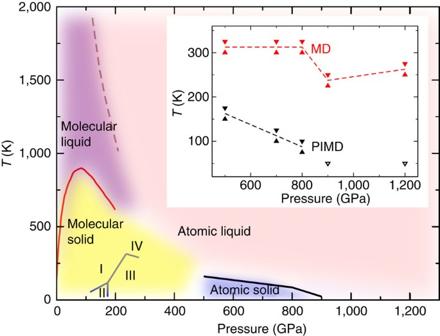Figure 2: Phase diagram of hydrogen. Regions of stability for the molecular solid (yellow), molecular liquid (purple), atomic solid (blue) and atomic liquid (pink) are indicated by the various colours. The dashed line separating the molecular and atomic liquid phases is taken from quantum Monte Carlo calculations35. The solid line separating the molecular solid and molecular liquid phases is taken fromab initioMD simulations36, whose negative slope has been confirmed by experiment6. The thick black line is the melting curve obtained in this study from theab initioPIMD coexistence simulations. The solid lines separating phases I, II, III and IV are from (refs12,13). The inset shows how the high-pressure melting curve (dashed lines) are established here. The black and red triangles (inset) correspond to the PIMD and MD results, respectively. The solid up triangles give the highest temperatures for solidification and the solid down triangles show the lowest temperatures for liquefaction. At 900 and 1,200 GPa, the so-called degeneracy temperature is ~40 K, below which the exchange of nuclei will be important. Accordingly, 50 K was the lowest temperature examined in our PIMD simulations. At this temperature each simulation yields a liquid state, and so the two open triangles at 900 and 1,200 GPa indicate upper bounds for the melting temperature. Figure 2: Phase diagram of hydrogen. Regions of stability for the molecular solid (yellow), molecular liquid (purple), atomic solid (blue) and atomic liquid (pink) are indicated by the various colours. The dashed line separating the molecular and atomic liquid phases is taken from quantum Monte Carlo calculations [35] . The solid line separating the molecular solid and molecular liquid phases is taken from ab initio MD simulations [36] , whose negative slope has been confirmed by experiment [6] . The thick black line is the melting curve obtained in this study from the ab initio PIMD coexistence simulations. The solid lines separating phases I, II, III and IV are from (refs 12 , 13 ). The inset shows how the high-pressure melting curve (dashed lines) are established here. The black and red triangles (inset) correspond to the PIMD and MD results, respectively. The solid up triangles give the highest temperatures for solidification and the solid down triangles show the lowest temperatures for liquefaction. At 900 and 1,200 GPa, the so-called degeneracy temperature is ~40 K, below which the exchange of nuclei will be important. Accordingly, 50 K was the lowest temperature examined in our PIMD simulations. At this temperature each simulation yields a liquid state, and so the two open triangles at 900 and 1,200 GPa indicate upper bounds for the melting temperature. Full size image The negative slope of the melting curve up to 800 GPa suggests that at even higher pressures a lower-temperature liquid phase might exist. Motivated by this, we carry out simulations at 900 and 1,200 GPa. However, in this pressure range we have to consider nuclear exchange effects, which are neglected in the PIMD simulations performed here, but which could potentially become significant. Indeed, analysis of our simulations reveals that at these pressures the dispersion of the beads in the path-integral ring polymer becomes comparable to the smallest interatomic separations when the temperature is below ~40 K (see Supplementary Figure S6 ). This is the so-called quantum degeneracy temperature below which the exchange of nuclei will be important, and consequently simulations with a (standard) PIMD approach are expected to be inaccurate. With this in mind we perform all simulations in this very high-pressure regime at T ≥50 K. Interestingly, we find that at 50 K, at both 900 and 1,200 GPa, the systems are already in the liquid state, revealing that the melting temperature at these pressures is <50 K. Whether the liquid phase is the 0 K ground state of hydrogen at these pressures is not something we can establish at this stage. However, the large negative slope of the melting curve at lower pressures and the observation of a liquid phase at temperatures as low as 50 K provide strong support for Ashcroft’s [16] low-temperature liquid metallic state of hydrogen, and it implies that any room temperature superconductor in this regime would have to be a liquid. It is instructive to compare the results of the ab initio PIMD simulations with those obtained from the ab initio MD approach in which the nuclei are approximated by classical point-like particles. To this end, we perform a second complete set of coexistence simulations with ab initio MD across the entire 500–1,200 GPa range. The ab initio MD melting curve is shown by the red data in the inset of Fig. 2 , where it can be seen that the melting temperatures obtained from the MD simulations are much higher than those from the fully quantum PIMD simulations. The ab initio MD melting temperature is well above 200 K across the pressure range 500–1,200 GPa, and the slope of the melting curve is small. A melting curve with a negative slope was also found above 90 GPa in the ab initio MD simulations of hydrogen by Bonev et al. [5] and above 10 GPa in lithium [37] . In the present study, ab initio MD simulations with classical nuclei exhibit considerably higher melting temperatures than the ab initio PIMD ones at pressures above 500 GPa, which shows that the quantum description of the protons strongly depresses the melting point. The entropy arising from the greater delocalization of the protons in the quantum description has a crucial role in stabilizing the low-temperature liquid. In conclusion, our results are consistent with a melting curve with a negative slope between an atomic solid and a low-temperature (50 K or below) metallic atomic phase. A comparison of the MD with PIMD results shows that the quantum nature of the nuclei is responsible for the large negative slope of the melting curve and the consequent existence of the low-temperature metallic liquid. A natural conclusion from this is that the phase diagram of hydrogen in the pressure regime considered should exhibit rather large isotope effects. It is not clear from our studies whether the liquid phase survives down to 0 K, and this needs to be studied using other methods. The occurrence of the I 4 1 / amd solid above about 500 GPa indicates that a molecular-to-atomic solid–solid phase transition must occur at lower pressures, which could be accessible to experiments in the near future. Electronic structures Density functional theory calculations with the Perdew-Burke-Ernzerhof exchange-correlation functionals were performed with the VASP code [38] . Projector-augmented wave potentials were used along with a 500-eV plane wave cutoff energy. A Monkhorst–Pack k -point mesh of spacing 2π × 0.05 Å −1 was used along with a unit cell that typically contained 200 atoms. Convergence tests with large unit cells and higher plane wave cutoff energies, as well as comparisons between Perdew-Burke-Ernzerhof and other exchange-correlation functionals, are reported in Supplementary Notes 1 and 2 ( Supplementary Figs S2 and S4 ). Molecular dynamics MD and PIMD simulations were of the ‘Born–Oppenheimer’ type within the canonical ensemble (constant volume and constant temperature) ensemble, using a Nosé–Hoover chain thermostat. A 0.5-fs time step was used and all simulations were run for at least 20,000 steps (10 ps). The PIMD simulations made use of a self-developed implementation of this method in VASP. 32 beads were used to sample the imaginary-time path integral at each temperature, as this was found to be the minimum number of beads needed to obtain reliable estimates of the melting temperature ( Supplementary Fig. S3 ). When calculating real-time atomic diffusion in the liquid phase using the adiabatic centroid MD method ( Fig. 1e ), a smaller time step of 0.05 fs was used after thermalization and 20,000 steps were used to characterize the atomic diffusion. For more details, please refer Supplementary Note 2 . Two-phase simulations In simulating the melting curve, we used the ab initio PIMD method in association with the two-phase simulation technique. This treatment allows the Gibbs free energy (including enthalpic and entropic contributions) at finite temperatures to be implicitly evaluated when the melting curve is established. We note, however, that quantitative estimations of enthalpy and entropy are not obtained with this approach, unlike alternative methods, such as thermodynamic integration [39] . In these coexistence simulations, each run was initiated from a structure comprising a solid I 4 1 / amd phase and a liquid phase obtained by selecting samples from earlier simulations at higher temperatures. To test the sensitivity of the results to the chosen starting structures, we performed simulations with several different uncorrelated liquid-phase structures and found that the results were independent of the starting liquid structure. The system was normally found to liquefy or solidify after about 1–2 ps and equilibrium was reached soon afterwards (see Supplementary Fig. S5 ). For more computational details, including those related to the relative static enthalpy between different candidate solid phases and the superconductivity ( Supplementary Figs S1, S7 and S8 ), please read Supplementary Notes 1, 2 and 3 . How to cite this article: Chen, J. et al. Quantum simulation of low-temperature metallic liquid hydrogen. Nat. Commun. 4:2064 doi: 10.1038/ncomms3064 (2013).